Structures of Pup ligase PafA and depupylase Dop from the prokaryotic ubiquitin-like modification pathway Pupylation is a posttranslational protein modification occurring in mycobacteria and other actinobacteria that is functionally analogous to ubiquitination. Here we report the crystal structures of the modification enzymes involved in this pathway, the p rokaryotic u biquitin-like p rotein (Pup) ligase PafA and the depupylase/deamidase Dop. Both feature a larger amino-terminal domain consisting of a central β-sheet packed against a cluster of helices, a fold characteristic for carboxylate-amine ligases, and a smaller C-terminal domain unique to PafA/Dop members. The active site is located on the concave surface of the β-sheet with the nucleotide bound in a deep pocket. A conserved groove leading into the active site could have a role in Pup-binding. Nuclear magnetic resonance and biochemical experiments determine the region of Pup that interacts with PafA and Dop. Structural data and mutational studies identify crucial residues for the catalysis of both enzymes. The pupylation pathway [1] , [2] , [3] has an important role during the intracellular persistence of Mycobacterium tuberculosis ( Mtb ). It supports resistance of this pathogen towards oxidative and nitrosative stress encountered inside the host macrophages [4] , [5] . Mtb kills 2 million people every year and, with the emergence of multi-drug-resistant strains, new therapeutic approaches are urgently needed. The molecular components of the pupylation pathway, therefore, are promising targets for drug development. Pupylation is a posttranslational protein-tagging system that marks target proteins for degradation by proteasomes in Mtb and other actinobacteria [1] , [2] . The pupylation gene locus also occurs sporadically in other bacterial lineages [6] , [7] . In analogy to ubiquitination, a small (60–70 residues), p rokaryotic u biquitin-like p rotein (Pup) is covalently attached to lysine residues of target proteins via an isopeptide bond [1] , [2] , [3] . Pup shares no structural homology with ubiquitin and is disordered in its free form [8] , [9] , [10] . Pup is recognized by the amino-terminal coiled-coil domains of the proteasomal ATPase Mpa [10] , [11] , leading to ATPase-driven unfolding of pupylated substrate proteins followed by degradation inside the proteasome [12] , [13] . Although functionally analogous to ubiquitination, pupylation occurs by a chemically distinct pathway [3] . In mycobacteria, pupylation involves the sequential action of two homologous but catalytically different enzymes. First, the enzyme Dop ( d eamidase o f P up) converts the C-terminal glutamine of Pup (PupQ) to a glutamate (PupE), thereby rendering it ligation-competent [3] . Then, the enzyme PafA ( p roteasome a ccessory f actor A ) catalyses the formation of an isopeptide bond between the side chain of PupE's C-terminal glutamate and the ε-amino group of a substrate lysine [3] , [14] . To carry out the respective reactions, both enzymes, which were bioinformatically classified as belonging to the carboxylate-amine ligase family [7] , use ATP as a cofactor, but only the Pup ligase PafA turns over ATP [3] . In addition to performing the deamidation of PupQ to PupE [3] , Dop has an important role as depupylase by removing Pup from modified lysine residues [15] , [16] . PafA catalyses a two-step reaction proceeding through a phosphorylated intermediate formed at the C-terminal glutamate of Pup before transfer of Pup to the substrate acceptor lysine [14] , [17] . The detailed reaction mechanism for Dop remains unknown. In this work, we present the crystal structures of the two enzymes involved in the pupylation/depupylation pathway. Biochemical analysis of PafA and Dop variants, designed on the basis of the molecular architecture of the active sites, provides mechanistic insight. We demonstrate that the C-terminal half of Pup interacts with Dop and PafA and propose that a conserved groove observed in both enzymes may bind this part of Pup, thereby placing Pup's C-terminal residue near the active site. Crystallization and structure determination We solved the crystal structures of full-length Dop (57 kDa) from Acidothermus cellulolyticus (Dop Acel ) and full-length PafA (54 kDa) from Corynebacterium glutamicum (PafA Cglu ). 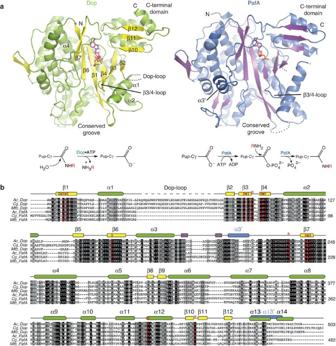Figure 1: Dop and PafA are close structural homologues. (a) The crystal structures of deamidase/depupylase Dop (green) fromA. cellulolyticuswith ATP and Pup ligase PafA (blue) fromC. glutamicumwith ADP. Front views are shown, looking into the β-sheet cradle (yellow for Dop and purple for PafA). The dotted lines indicate structurally undefined regions. Selected β-strands and α-helices are labelled in the Dop structure. Other structural features are indicated in both Dop and PafA. The catalysed reaction mechanism of Dop and PafA is depicted below the corresponding structures. (b) Schematic depiction of secondary structure elements above the amino-acid sequence alignments of Dop and PafA fromA. cellulolyticus,C.glutamicumandM.tuberculosis, respectively. The backbone is indicated by a grey line, linking α-helices (green, α1-14) and β-strands (yellow, β1-12) common to both enzymes, whereas differing structural elements in PafA are indicated as purple β-strands or blue α-helices, respectively. Backbone regions not visible in the structures are shown as dashed grey lines. The structure of Dop was solved by multiple isomorphous replacement and refined to a resolution of 2.6 Å without ATP and 2.85 Å with ATP ( Table 1 ). The final electron density map showed continuous density except for a disordered region between residues 36 to 80. The structure of PafA with ADP bound was solved by molecular replacement using the Dop structure and refined to a resolution of 2.15 Å ( Table 1 ). Table 1 Data collection and refinement statistics. Full size table PafA crystals contain two molecules per asymmetric unit, forming a stable dimer by swapping of the N-terminal strand-helix motif (β1 and α1, Supplementary Fig. S1 ). However, the position of the exchanged strand and helix is equivalent to the position of the corresponding strand and helix in the monomer, based on comparison with the structure of Dop. Therefore, the PafA structure is displayed and discussed throughout this manuscript as the catalytically active monomer (chain A: N52-A477 and chain B: S2-S51). Dop and PafA feature two tightly interacting domains Dop Acel and PafA Cglu (38% sequence identity) are globular proteins with high structural homology ( Fig. 1 ), reflected in a low r.m.s.d. value of 2.12 Å for the superimposition of equivalent Cα atoms (396 aligned Cα, Supplementary Fig. S2 ). In both structures, two tightly interacting domains can be distinguished. The larger N-terminal domain comprising roughly the first 400 residues (PafA: 410, Dop: 425) is structurally related to carboxylate-amine ligases. In both Dop and PafA, this domain features a twisted central β-sheet of six β-strands (β1-4, β6, β7) in anti-parallel orientation forming a concave surface referred to here as the β-sheet cradle, which is surrounded by a cluster of helices on the convex backside of the sheet. Loops, extending from the C- and N-terminal ends of the β-strands, cover part of the concave face of the sheet, closing off one end. The opposite end is open, with a well-defined groove that is lined with conserved residues leading away from the β-sheet cradle ( Fig. 1a ). The small C-terminal domain of about 70 residues is formed by a short, three-stranded β-sheet (β10-12) packed against two (PafA; α12, α13′) or three (Dop; α12, α13, α14) short helices. This domain is not found in other carboxylate-amine ligases and thus presents a structural feature unique to the Dop/PafA family. Figure 1: Dop and PafA are close structural homologues. ( a ) The crystal structures of deamidase/depupylase Dop (green) from A. cellulolyticus with ATP and Pup ligase PafA (blue) from C. glutamicum with ADP. Front views are shown, looking into the β-sheet cradle (yellow for Dop and purple for PafA). The dotted lines indicate structurally undefined regions. Selected β-strands and α-helices are labelled in the Dop structure. Other structural features are indicated in both Dop and PafA. The catalysed reaction mechanism of Dop and PafA is depicted below the corresponding structures. ( b ) Schematic depiction of secondary structure elements above the amino-acid sequence alignments of Dop and PafA from A. cellulolyticus , C . glutamicum and M . tuberculosis , respectively. The backbone is indicated by a grey line, linking α-helices (green, α1-14) and β-strands (yellow, β1-12) common to both enzymes, whereas differing structural elements in PafA are indicated as purple β-strands or blue α-helices, respectively. Backbone regions not visible in the structures are shown as dashed grey lines. Full size image Nucleotide binding to Dop and PafA The active site of both enzymes is located in the β-sheet cradle ( Fig. 1 ). The adenine moiety is buried deeply in a mostly hydrophobic pocket formed by β1 and β6 on one side and a highly conserved loop preceding β7, as well as loops emanating from the C-terminal domain on the other side ( Fig. 2 ). A conserved arginine at the beginning of the C-terminal domain (R433 in Dop, R418 in PafA) interacts with the adenine ring. A conserved tryptophan (W453 in Dop, W440 in PafA) in the loop between β10 and β11 flanks the adenine pocket and contacts the sugar moiety ( Fig. 2b ). Supporting the importance of this interaction, mutating W440 of PafA to alanine prevents conjugation of PupE (a PupQ64E variant) to the known target protein PanB [18] (ketopantoate hydroxymethyltransferase) ( Fig. 3a ). 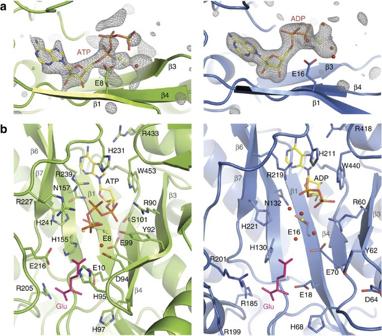Figure 2: Active site of Dop and PafA. (a) The Fo–Fc map of the Dop:ATP density contoured at 2.5 σ and PafA:ADP contoured at 3.0 σ shows the location of ATP or ADP binding, respectively. The unbiased Fo–Fc difference Fourier map was calculated by simulated annealing using a model, in which ADP or ATP, Mg2+and water molecules were omitted. Strands β1, β3 and β4, as well as glutamate E8 (Dop) or E16 (PafA) are depicted. (b) Zoomed view of the Dop (left) and PafA (right) active site. Important residues are shown in stick representation. Bound Mg2+ions are shown as yellow spheres, bound water molecules as red spheres. A glutamate molecule (pink) has been placed into the active site according to its equivalent position in the glutamate cysteine ligase structure (PDB: 2GWD). Figure 2: Active site of Dop and PafA. ( a ) The Fo–Fc map of the Dop:ATP density contoured at 2.5 σ and PafA:ADP contoured at 3.0 σ shows the location of ATP or ADP binding, respectively. The unbiased Fo–Fc difference Fourier map was calculated by simulated annealing using a model, in which ADP or ATP, Mg 2+ and water molecules were omitted. Strands β1, β3 and β4, as well as glutamate E8 (Dop) or E16 (PafA) are depicted. ( b ) Zoomed view of the Dop (left) and PafA (right) active site. Important residues are shown in stick representation. Bound Mg 2+ ions are shown as yellow spheres, bound water molecules as red spheres. A glutamate molecule (pink) has been placed into the active site according to its equivalent position in the glutamate cysteine ligase structure (PDB: 2GWD). 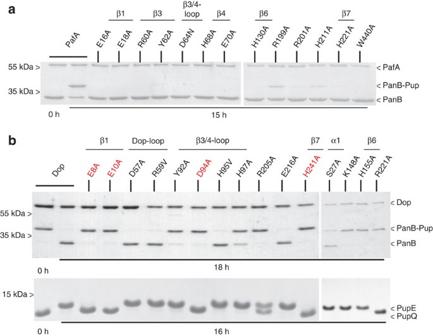Figure 3: Structure-based active site variants of Dop and PafA. (a) Formation of a covalent PanB-Pup conjugate analysed by SDS–PAGE and Coomassie staining after incubation of PanBMtb(6 μM) and PupECglu(16 μM) with PafACglu(1 μM) in the presence of ATP (5 mM). (b) Depupylation of a covalent PanB-Pup conjugate (upper gel) and deamidation of PupQ (lower gel) by Dop after incubation of PanBMtb-PupEAcel(2 μM) or PupEAcel(25 μM), respectively, with DopAcel(0.5 μM) in the presence of ATP (5 mM). Variants, fully inactive for both depupylation and deamidation, are depicted in red. Full size image Figure 3: Structure-based active site variants of Dop and PafA. ( a ) Formation of a covalent PanB-Pup conjugate analysed by SDS–PAGE and Coomassie staining after incubation of PanB Mtb (6 μM) and PupE Cglu (16 μM) with PafA Cglu (1 μM) in the presence of ATP (5 mM). ( b ) Depupylation of a covalent PanB-Pup conjugate (upper gel) and deamidation of PupQ (lower gel) by Dop after incubation of PanB Mtb -PupE Acel (2 μM) or PupE Acel (25 μM), respectively, with Dop Acel (0.5 μM) in the presence of ATP (5 mM). Variants, fully inactive for both depupylation and deamidation, are depicted in red. Full size image The tri-phosphate chain of ATP in Dop extends along the β-sheet cradle with the γ-phosphate pointing towards the putative glutamate-binding site. The di-phosphate chain of ADP in the active site of PafA adopts a different conformation that potentially represents the state after ATP cleavage. The β-sheet cradle in both enzymes is lined by conserved residues holding the nucleotide in place ( Fig. 2b ; Supplementary Table S1 ). In Dop, the charges of the α-, β- and γ-phosphates are neutralized by two arginines (R227 and R239) located in the loop preceding β7 ( Fig. 2b ) and a third one in strand β3 (R90 in Dop, R60 in PafA). Underlining the importance of this interaction, PafA variant R60A is unable to ligate PupE to PanB. R239 and an equivalent arginine in PafA (R219) also contribute to binding of the adenine moiety of the nucleotide through hydrophobic stacking contacts. In PafA, the α-phosphate is contacted by H211 ( Fig. 2b ) and, consequently, mutation of this residue to an alanine (H211A) leads to reduced activity ( Fig. 3a ). Furthermore, a conserved glutamate residue in β1 (E8 in Dop, E16 in PafA) coordinates two Mg 2+ ions in Dop (n2 and n3) and one in PafA (n2), which, in turn, coordinate the phosphates ( Fig. 2 ). This conserved glutamate is part of an ATP-binding motif shared by all members of the carboxylate-amine ligase family ( Supplementary Fig. S3 and Supplementary Table S1 ). On the basis of homology with other carboxylate-amine ligases [19] , [20] , the second conserved glutamate in this motif (E10 in Dop, E18 in PafA) is expected to coordinate an additional Mg 2+ ion (n1) that is not occupied in our crystal structures likely due to the absence of a bound substrate (Pup). Alanine substitution of either of these residues (E8A and E10A) renders Dop unable to perform the deamidation and depupylation reaction ( Fig. 3b ) and PafA (E16A and E18A) unable to catalyse the ligation ( Fig. 3a ). An additional glutamate (E99 in Dop, E70 in PafA) located in strand β4 also contributes to coordination of the Mg 2+ ions, either directly (Dop) or via a water molecule (PafA). Two histidine residues on strands β6 and β7 (H155 and H241 in Dop; H130 and H221 in PafA) coordinate the Mg 2+ ion in position n2 in the Dop structure. Changing either one of these residues to an alanine abolishes depupylation in Dop (H155A or H241A) and ligation in PafA (H130A or H221A). Deamidation by Dop, however, can still occur in the case of the Dop variant H155A ( Fig. 3b ). Active site features of PafA and Dop The putative binding site for Pup's C-terminal glutamate residue is located at the accessible end of the β-sheet cradle, close to the N-terminal end of β6, based on the location of the glutamate molecule in the structure of glutamine synthetase [19] ( Fig. 2b ; Supplementary Fig. S3 ). A conserved arginine serves to coordinate the α-carboxylate group of glutamate in glutamine synthetase [20] . PafA and Dop have an equivalent arginine residue (R205 in Dop, R185 in PafA) in the same location ( Fig. 2b ; Supplementary Fig. S3 and Supplementary Table S1 ), which is likely to help position the C-terminal residue of Pup in the active site. In Dop, changing this residue to an alanine (R205A) impairs depupylation and significantly slows deamidation ( Fig. 3b ). The mechanism of Dop and PafA differs particularly in one aspect: PafA must activate the γ-carboxylate in the C-terminal glutamate of Pup through formation of a phosphorylated intermediate. This is necessary, because the hydroxide anion is a poor leaving group. Deamidation or depupylation on the other hand can proceed without such activation, because ammonium or substituted amines are much better leaving groups. PafA forms a surprisingly stable phosphorylated Pup intermediate, where the γ-phosphate of ATP has been transferred to the γ-carboxylate of Pup's C-terminal glutamate [17] . In contrast, the amide group of the γ-carboxamide of Pup's C-terminal Gln is a very poor nucleophile and could only serve this function under very special steric circumstances (for example, when forced by enzyme constraints into a sp3 hybridization state [21] ). It is therefore not expected to attack the γ-phosphate of ATP, which is in agreement with the observation that Dop does not hydrolyse ATP [3] . The inability of Dop to support attack of the carboxylate oxygen of the PupE deamidation product on the γ-phosphate of ATP might be caused by a different relative positioning between the γ-carboxylate of Pup's C-terminal Glu residue and the γ-phosphate of ATP. Alternatively, ATP might not remain bound in the active site, once the product has been formed and could be required to rebind after PupE has been released. Although Dop and PafA catalyse different reactions, parts of the mechanism are expected to require similar catalytic assistance. In both reactions, a nucleophilic attack must occur on the carbonyl-carbon of the C-terminal glutamine/glutamate side chain of Pup. This attack would be facilitated by active site residues acting as a catalytic base (H-acceptor) to activate the nucleophile, which in the case of Dop is water and in case of PafA the ε-amino group of lysine. The ε-amino group of the target lysine is expected to be located in a position equivalent to the ammonium ion-binding site in glutamine synthetase [20] , where residues in the loop between strands β3 and β4 coordinate the nucleophile. On the basis of their position in the active site and their chemical properties, possible candidates for proton abstraction in PafA are D64 or H68 in the β3/4-loop ( Fig. 2b ). Although in PafA, these residues are part of a flexible loop and point away from the active site, amino-acid substitutions at these positions (D64N or H68A) result in pupylation-inactive (D64N) and only marginally active (H68A) variants of PafA ( Fig. 3a ). The equivalent loop in Dop adopts a closed conformation bringing D94 and H97 towards the active site. The Dop variant D94A is completely inactivated, while the H97A variant is still able to deamidate PupQ and exhibits some depupylation activity ( Fig. 3b ). This suggests that the catalytic bases supporting nucleophilic attack by the ε-amino group and by water in PafA and Dop are D64 and D94, respectively, whereas the conserved histidine residue may have a role in binding and positioning of Pup in the active site. This would also agree with the fact that in Dop, the aspartate is located close to the putative position of the glutamate γ-carboxylate, although the histidine is located farther away. The nucleophilic attack could be further supported by coordination of the carbonyl oxygen to a positively charged side chain of the enzyme, resulting in a more electrophilic carbonyl-carbon in the C-terminal Pup glutamine/glutamate side chain. In PafA, this role could be played by one of the arginine side chains located above the putative glutamate-binding site following the α3′-helix, R199 or R201. Alanine variants at this position in PafA exhibit marginal (R201A) or reduced (R199A) ligase activity ( Fig. 3a ). Because the second arginine (R201) is also conserved in Dop (R221) and an alanine mutation of that residue (R221A) leads to inactivity as well ( Fig. 3b ), it is the more likely candidate for this role. Unique features of Dop compared with PafA To identify residues that specifically act in deamidation/depupylation, we looked for residues or sequence stretches present or conserved only in Dop but not in PafA ( Supplementary Fig. S4 ). One such region is the loop preceding strand β2 in Dop, termed the Dop-loop. Unexpectedly, deletion of this loop from Dop results in a Dop variant (Dop ΔDop-loop ) that still shows full deamidase and PanB-Pup depupylase activity ( Supplementary Fig. S4c ). Removal of this Dop-specific loop also did not convert Dop into a ligase, because Dop ΔDop-loop was unable to modify PanB with Pup ( Supplementary Fig. S4d ). Additionally, three residues that are strictly conserved in Dop, but not in PafA, were identified: S27, H95 and K148. We produced variants replacing these residues individually with the respective residues found in PafA from the same organism ( A . cellulolyticus ). Two of these variants, S27A and H95 V, exhibited wild-type behaviour. The variant K148A could no longer carry out depupylation of PanB-Pup, but was still deamidation-active ( Fig. 3b ). Significant differences between Dop and PafA are also observed in the region between helix α3 and strand β7 (Dop Acel : 208–216, PafA Acel : 174–182). In PafA, this region is more structured, forming an additional α-helix (α3′). Swapping this region in Dop with the equivalent stretch of sequence from PafA Acel , created the variant Dop α3′PafA ( Supplementary Fig. S4 ). Dop α3′PafA was still able to deamidate PupQ and depupylate PanB-Pup in vitro . Even when this sequence swap was combined with deletion of the Dop-loop to form Dop ΔDop-loop-α3′PafA , no effect on these two activities was observed in comparison to wild-type Dop. The short loop segment between strands β3 and β4 (β3/4-loop) adopts a different conformation in Dop and PafA. A Dop variant, wherein this region was replaced with the equivalent region of PafA, Dop β3/4-loop-PafA , could still deamidate, but could not depupylate PanB-Pup ( Supplementary Fig. S4 ). Two alanine-substituted Dop variants in this region (Y92A and H97A) showed similar behaviour ( Fig. 3b ), a defect in depupylation but not deamidation. To exclude a concentration-dependent effect, we repeated the depupylation assay with the same concentration of PanB-Pup as used for PupQ in deamidation and still observed that depupylation was impaired for the variants in comparison with wild type ( Supplementary Fig. S5 ). This suggests that this region of Dop has a role in controlling accessibility to the isopeptide bond or in binding the target protein portion (in this case PanB) of pupylated substrates. Binding of Pup to Dop and PafA Dop and PafA catalyse distinct reactions in the pupylation pathway [3] , [15] , [16] . However, both must recognize and bind Pup. We performed a gel-based pupylation assay in combination with electrospray ionisation mass spectrometry using C-terminal PupE fragments of varying lengths. PupE 38-64 was identified as the shortest peptide fragment tested that can still be attached to PanB by PafA ( Fig. 4a ; Supplementary Fig. S6 ). Having established residues 38–64 of Pup as sufficient for conjugation by PafA, we determined the residues of Pup involved in binding to both enzymes using nuclear magnetic resonance (NMR). Considering the high degree of sequence conservation in residues 38–64 of Pup, NMR titrations with 15 N-labelled PupE Mtb or PupQ Mtb were performed with PafA from Bifidobacterium angulatum (PafA Bang ) and Dop from C . glutamicum ( Dop Cglu ), which both exhibited sufficient solubility unlike their Mtb homologues. Titrations were monitored in 15 N- 1 H correlation spectra after addition of the unlabelled enzymes ( Fig. 4b ). Resonance positions of Pup signals are insensitive to the addition of Dop, whereas the intensity of specific signals gradually decreased with increasing amounts of Dop added ( Fig. 4b ; Supplementary Fig. S7 ), indicating slow exchange on the NMR timescale. This is consistent with a submicromolar affinity of Dop for Pup measured by isothermal titration calorimetry (ITC) ( Supplementary Fig. S8 ). Pup signal positions showed more significant chemical shift changes when titrated with PafA and rapidly decreased in intensity at very low ratios of enzyme to Pup indicating that the complex is in intermediate exchange on the NMR timescale ( Fig. 4b ; Supplementary Fig. S7 ). This is consistent with the micromolar affinity measured for the Pup–PafA complex ( Supplementary Fig. S8 ). 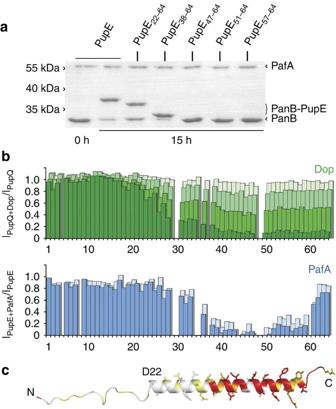Figure 4: Interaction of Dop and PafA with Pup. (a) Gel-based PanBMtbpupylation assay using C-terminal PupE fragments of varying size. Formation of covalent conjugates between PanBMtband the indicated Pup-fragments analysed by Coomassie-stained SDS–PAGE after incubation of PanBMtb(6 μM) and corynebacterial Pup-fragments (16 μM) with PafACglu(1 μM) in the presence of ATP (5 mM). (b) Binding of PupQMtbto DopCgluat ratios of 1:0.1, 1:0.2, 1:0.5 and 1:1 (in increasingly dark shades of green) or PupEMtbto PafABangat ratios of 1:0.1 and 1:0.25 (light and dark blue, respectively) analysed by NMR. Relative peak heights of backbone resonances from assigned residues in [15N,1H]-HSQC or [15N,1H]-HMQC spectra recorded at each ratio of Pup to enzyme were determined by normalizing to their intensity in the spectrum of Pup alone, resulting in a 'footprint' on the Pup sequence indicating the area of interaction. (c) Structural model of Pup generated with Modeller using PDB entry 3m91 (ref.11) and helical restraints for residues 52 to 60 coloured according to residue conservation. High conservation is indicated by red, low conservation by white. The model is approximately aligned to the residue numbers in panelb. Figure 4: Interaction of Dop and PafA with Pup. ( a ) Gel-based PanB Mtb pupylation assay using C-terminal PupE fragments of varying size. Formation of covalent conjugates between PanB Mtb and the indicated Pup-fragments analysed by Coomassie-stained SDS–PAGE after incubation of PanB Mtb (6 μM) and corynebacterial Pup-fragments (16 μM) with PafA Cglu (1 μM) in the presence of ATP (5 mM). ( b ) Binding of PupQ Mtb to Dop Cglu at ratios of 1:0.1, 1:0.2, 1:0.5 and 1:1 (in increasingly dark shades of green) or PupE Mtb to PafA Bang at ratios of 1:0.1 and 1:0.25 (light and dark blue, respectively) analysed by NMR. Relative peak heights of backbone resonances from assigned residues in [ 15 N, 1 H]-HSQC or [ 15 N, 1 H]-HMQC spectra recorded at each ratio of Pup to enzyme were determined by normalizing to their intensity in the spectrum of Pup alone, resulting in a 'footprint' on the Pup sequence indicating the area of interaction. ( c ) Structural model of Pup generated with Modeller using PDB entry 3m91 (ref. 11 ) and helical restraints for residues 52 to 60 coloured according to residue conservation. High conservation is indicated by red, low conservation by white. The model is approximately aligned to the residue numbers in panel b . Full size image The interaction of PafA with Pup results in a footprint spanning residues 36 to 60 of Pup. The interaction profile of Dop on Pup is somewhat wider, extending from residues ~28 to 64. These data also suggest that in PafA, the four C-terminal residues of Pup are less constrained than in Dop, which agrees with the more narrow shape of the active site cradle in the putative glutamine-/glutamate-binding region in Dop. The NMR experiments indicate that both Dop and PafA bind to the conserved C-terminal half of Pup, whereas the N-terminal half does not participate. The interacting stretch of residues overlaps with a region of Pup that has previously been predicted to have a propensity for forming coiled-coils [7] , [10] and adopts a helical conformation when bound to the proteasomal ATPase Mpa [11] ( Fig. 4c ). It is possible that Pup may also adopt a helical conformation when it is bound by Dop or PafA. Surface representations of Dop and PafA, coloured according to residue conservation, reveal a conserved groove leading into the active site where the glutamate is bound in glutamine synthetases [19] , [20] ( Fig. 5a,b ). Pup could bind this groove either in an extended or a helical conformation. The mutation of L376E in PafA near this groove abolishes Pup ligation activity ( Supplementary Fig. S9a ). In Dop, mutations that introduce a negatively charged residue (Q139E or R400E) in this conserved groove strongly impair binding of PupQ as tested by analytical gel filtration and abrogate depupylation of PanB-Pup ( Supplementary Fig. S9bc ). These results are consistent with a putative role of the groove in Pup binding. 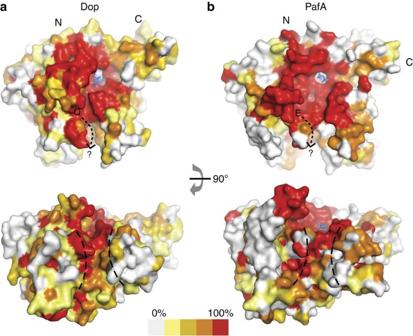Figure 5: Conserved surface representation of Dop and PafA. (a) Deamidase/depupylase Dop. (b) Pup ligase PafA. Highly conserved residues are outlined in red, nonconserved residues in white. Nucleotides are shown in stick representation (blue). Termini of the polypeptide chains are depicted with either N or C, respectively. The potential Pup-binding groove (indicated by black dotted lines in the lower panels) shows intermediate to high conservation. Figure 5: Conserved surface representation of Dop and PafA. ( a ) Deamidase/depupylase Dop. ( b ) Pup ligase PafA. Highly conserved residues are outlined in red, nonconserved residues in white. Nucleotides are shown in stick representation (blue). Termini of the polypeptide chains are depicted with either N or C, respectively. The potential Pup-binding groove (indicated by black dotted lines in the lower panels) shows intermediate to high conservation. Full size image Pupylation is an ubiquitin-like modification that has evolved in a subset of bacteria, amongst them the highly pathogenic M . tuberculosis ( Mtb ) [1] , [2] . Persistence of Mtb in the host is supported by this tagging pathway [5] , making it interesting from a medical perspective. The molecular details of the Pup modification system are also interesting from a mechanistic point of view, because pupylation occurs by a pathway chemically distinct from ubiquitination [3] . To provide the molecular framework for the mechanism of pupylation, we have determined the X-ray structures of both the Pup ligase PafA and the depupylase/deamidase Dop. Structural alignment of Dop with PafA shows that the two enzymes are similar in overall structure and fold with differences occurring in loop regions between the central β-sheet and the helix cluster packed against the convex side of the sheet ( Fig. 1a ; Supplementary Figs S2 and S4 ). The active site is located in a broad β-sheet cradle accessible at one end ( Fig. 1a ). The ATP binding site, situated in both enzymes at the closed end of the β-sheet cradle, is well shielded from solution ( Figs 1a and 2 ). This is achieved at least in part by the small, C-terminal domain, in addition to the adjacent loop preceding strand β7. Because of this arrangement, the nucleobase and the ribose of the nucleotide are completely buried and only the phosphates are exposed. On the basis of their bioinformatic classification as carboxylate-amine ligases, PafA and Dop were both predicted to act as Pup ligases [7] . However, despite the high homology between Dop and PafA, biochemical analysis clearly established distinct enzymatic activities for PafA and Dop, with PafA acting canonically in isopeptide-bond formation whereas Dop surprisingly provides the opposing peptidase/deamidase activity [3] , [15] , [16] . There are several differences in the molecular architecture of both enzymes potentially contributing to the distinct enzyme activities ( Supplementary Fig. S4 ). One obvious difference is a flexible region with multiple conserved residues downstream of helix α1, which is present only in Dop members (Dop-loop, Fig. 1b ). Although it is disordered in our structure, this region could become more ordered in the presence of substrates or could have a role in the interaction with other potential binding partners. Another major difference between the two enzymes occurs in the region between helix α3 and strand β7. In PafA, this region is more conserved, and our structures show that it contains two short β-strands and one short α-helix in PafA (α3′), whereas in Dop it is less structured. This region flanks and partially covers the putative glutamyl residue-binding region and could, therefore, contribute to substrate binding and positioning of the Pup C-terminal end. Furthermore, the β3/4-loop in Dop seems more rigid than in PafA and could constrain the accessibility of the active site and also influence the positioning of Pup's C-terminus. Interestingly, the exchange of any of these regions in Dop with the analogous parts of PafA does not abolish the ability of Dop to depupylate/deamidate substrates in vitro and, more importantly, it does not lead to a gain of function allowing pupylation to be carried out by Dop ( Supplementary Fig. S4 ). This excludes each of these structural elements as a single determining factor for Dop activity. The deamidated form of Pup (PupE) is generated as a product of both the deamidation and the depupylation reaction. However, the carboxylate oxygen of the PupE product in Dop is apparently unable to attack the γ-phosphate of ATP. This might be caused by a different positioning of this carboxylate with respect to the γ-phosphate of ATP, preventing close enough approach or, alternatively, by asynchronous binding of PupE and ATP. A common feature of the pupylation/depupylation enzymes is a conserved groove running along the surface of the large domain and into the β-sheet cradle ( Fig. 5 ). It leads directly to the site where in homologous ligase structures the glutamate substrate is bound [19] . Essential features of this glutamate-binding site are conserved in Dop and PafA. For example, in the case of glutamine synthetase, the conserved arginine (R321) is involved in binding of the α-carboxylate of glutamate [20] . The same residue is also present in the corresponding position in Dop (R205) and PafA (R185) ( Fig. 2b ; Supplementary Table S1 and Supplementary Fig. S3cd ), indicating that both Dop and PafA probably bind Pup's C-terminal glutamine/glutamate at the same position. The dimensions of the conserved groove and the fact that it leads towards the putative glutamyl binding site, makes it an intriguing possibility that Pup might bind in the groove with its C-terminal residue positioned close to the β-sheet cradle. Although free Pup was shown to be mostly disordered [8] , [9] , [10] , the C-terminal part of Pup adopts an α-helical structure on binding to the proteasomal ATPase Mpa [10] , [11] . Hence, the C-terminal half of Pup, identified by NMR and biochemical experiments as interacting with Dop and PafA, could also bind in the groove in a helical conformation. As this region of Pup overlaps in part with the interaction site for Mpa [10] , [11] , the depupylase Dop and Mpa are likely to be sterically prevented from binding Pup simultaneously, and thus they compete for pupylated substrates, ultimately exerting influence on the fate of the substrate as degradation or depupylation target. It is interesting that Dop variants with changes in the β3/4 strand region are capable of catalysing deamidation but are impaired in depupylation. This region of Dop might be involved in binding of the target protein portion of the pupylated substrate or act to control access to the isopeptide bond. Proteomic studies have shown that the Pup ligase PafA has a large array of target proteins of varying size, oligomeric state and fold [22] , [23] . Similarly, the depupylase Dop was shown to remove Pup from numerous pupylated targets [15] , [16] . This promiscuity and low selectivity is reflected in a rather open approach to the active site allowing easy access of protein substrates from the concave face of the β-sheet cradle. Dop and PafA are both strictly required for pupylation in mycobacteria [2] , [3] , [24] , and thus represent attractive targets for drug development. On the basis of the presented structural data, potential target sites are the Pup-binding groove or the nucleotide-binding pocket. The nucleotide-binding pocket has unique features for PafA/Dop members of the carboxylate-amine ligase family because of the contribution of the C-terminal domain. Both targets are thus expected to be specific to the pupylation pathway, so that compounds binding to them should not inhibit other members of this family. The structural and biochemical data presented here provide a framework for future mechanistic experiments on the pupylation pathway. Cloning To produce A . cellulolyticus Dop for crystallization experiments, the dop gene was amplified from genomic DNA of Acidothermus cellulolyticus ATCC 43068 and cloned with a C-terminal TEV-EGFP-His 6 tag via NdeI/EcoRI into a modified pET-vector (Novagen), resulting in the expression of a Dop Acel -TEV-EGFP-His 6 fusion protein. This construct was used to generate the Dop variants Dop ΔDop-loop , Dop α3′PafA , Dop ΔDop-loop-α3′PafA and Dop β3/4-loop-PafA via fusion PCR by exchanging the selected DNA sequence from Dop Acel with the targeted PafA Acel sequence (primer sequences are provided in Supplementary Table S2 ). For all other studies in this work, a variant of Dop Acel was generated in a modified pET-vector (Novagen) lacking the last two amino acids of the wild-type sequence and carrying a C-terminal His 5 -tag resulting in the dopΔGR-His 5 expression vector. Mutations of this gene were introduced by site-directed mutagenesis according to manufacturer's instructions (Stratagene). To prepare PafA protein used in the NMR study, the pafA gene from Bifidobacterium angulatum DSM 20098 was amplified from genomic DNA via PCR. Cloning was performed with a C-terminal TEV-EGFP-His 6 tag via NdeI/EcoRI into a modified pET-vector (Novagen), resulting in the expression of a PafA Bang -TEV-EGFP-His 6 fusion protein. All corynebacterial genes were generated by PCR from Corynebacterium glutamicum ATCC 13032 genomic DNA in a previous study [16] . The gene for PupE Acel was obtained from genomic DNA of Acidothermus cellulolyticus ATCC 43068 as described for the mycobacterium constructs [3] . Similarly, the PupQ Acel variant was obtained by using a modified reverse primer encoding a terminal glutamine. Expression and purification of proteins Dop Acel was expressed in Escherichia coli Rosetta (DE3) cells (Invitrogen) and PafA Bang was expressed in E. coli BL21 (DE3) (Invitrogen) from IPTG-inducible plasmids at 25 °C. Both were expressed as Dop Acel -TEV-EGFP-His 6 or PafA Bang -TEV-EGFP-His 6 fusion proteins and purified by Ni-affinity chromatography (HiTrap IMAC HP, GE Healthcare). After cleavage of the fusion protein with TEV-protease (Invitrogen), EGFP-His 6 and TEV-protease were removed by Ni-affinity chromatography. The same protocol was used to produce the variants Dop ΔDop-loop , Dop α3'PafA , Dop ΔDop-loop-α3'PafA and Dop β3/4-loop-PafA . PafA Bang was further purified by size-exclusion-chromatography on a Superdex200 column (GE Healthcare) in 25 mM Tris–HCl, pH 7.5, 300 mM NaCl and 5 mM 2-mercaptoethanol. The final size exclusion chromatography for Dop Acel was performed in 20 mM Tris–HCl, pH 7.5, 300 mM NaCl and 5 mM 2-mercaptoethanol. The DopΔGR-His 5 from A . cellulolyticus and PafA Cglu were expressed and purified as described [16] . Briefly, the proteins were expressed in E. coli Rosetta cells from an IPTG-inducible plasmid at 23 °C and were purified by Ni-affinity chromatography and subsequent size-exclusion-chromatography. The final size exclusion chromatography for all wild-type Dop Acel and variants of Dop Acel was performed on a Superdex200 column in 50 mM Tris–HCl, pH 7.5, 300 mM NaCl and 5 mM 2-mercaptoethanol. The generated Dop variants all elute at the same retention volume as the wild-type protein. For crystallization of PafA Cglu , the final gel filtration step was performed on a Superose6 column in 20 mM Tris–HCl, pH 7.5, 50 mM NaCl and 5 mM DTT. For biochemical experiments with wild-type PafA C glu and variants of PafA Cglu , the final gel-filtration step was performed on a Superdex75 column in 50 mM Tris–HCl, pH 7.5, 300 mM NaCl, 20 mM MgCl 2 and 1 mM DTT. The generated PafA variants all elute at the same retention volume as the wild-type protein. PanB Mtb -His 6 was purified using Ni 2+ NTA affinity chromatography, as described [3] . Pup Acel , full-length Pup and Pup 22–64 from C. glutamicum were expressed and purified as described previously [3] . Other corynebacterial Pup truncations were synthesized (GeneScript). All protein concentrations were determined spectrophotometrically. 15 N-labelled Pup from M . tuberculosis H37Rv was produced by growing the cells in M9 minimal medium supplemented with 15 N (98%) ammonium chloride obtained from Cambridge Isotope Laboratories or Sigma-Aldrich and purified as described [3] , [14] . For NMR studies, cell lysis and Ni-affinity purification were performed in 50 mM Na 2 HPO 4 , pH 7.8 and 300 mM NaCl followed by gel filtration on a Superose75 column in 20 mM Na 2 HPO 4 , pH 6.0 and 50 mM NaCl and then exchanged into the final NMR buffer using centricon concentrators. Deamidation assay PupQ Acel (25 μM) was incubated with 0.5 μM Dop in reaction buffer (50 mM Tris–HCl, pH 7.5 (23 °C), 150 mM NaCl, 10% Glycerol, 1 mM DTT, 20 mM MgCl 2 ) supplemented with 5 mM ATP at 30 °C for 16 h as described in ref. 3 . The formation of PupE was analysed by SDS–PAGE and Coomassie staining. Pup-conjugation assay C. glutamicum Pup variants (Pup 57-64 , Pup 51–64 , Pup 47–64 , Pup 38–64 , Pup 22–64 or full-length PupE; 16 μM) were incubated with 6 μM PanB Mtb and 1 μM PafA Cglu in reaction buffer (50 mM Tris–HCl, pH 7.5 (23 °C), 300 mM NaCl, 10% Glycerol, 1 mM DTT, 5 mM MgCl 2 ) supplemented with 5 mM ATP at 23 °C for 15 h as described in ref. 3 . The formation of covalent PanB-Pup conjugates was analysed by SDS–PAGE and electrospray ionisation mass spectrometry. Depupylation assay PanB Mtb -Pup Acel conjugate (2 μM or 25 μM) (produced as described in ref. 16 ) was incubated with 0.5 μM Dop at 30 °C for 18 h in reaction buffer (50 mM Tris–HCl, pH 7.5 (23 °C), 150 mM NaCl, 10% Glycerol, 1 mM DTT, 20 mM MgCl 2 ) supplemented with 5 mM ATP. The formation of PanB Mtb and PupE Acel was analysed by SDS–PAGE and Coomassie staining. Crystallization and derivatization Purified Dop Acel was supplemented with 20 mM MgCl 2 , 5 mM 2-mercaptoethanol and 3 mM ATP. Crystallization was carried out in sitting-drop vapour diffusion plates at a protein concentration of 15 mg ml −1 at 26 °C. Samples were mixed with an equal volume of reservoir solution (0.1 M HEPES-HCl, pH 7.2, and 14% (v/v) PEG-3350). Before flash freezing, the crystals were stabilized by increasing the PEG concentration by 1–3% (v/v) and adding ethylene glycol to a final concentration of 20% (v/v). Soaking of Dop crystals with ATP was performed in cryo-stabilization solution with 5 mM ATP for 30 min. Crystals were derivatized in cryo-stabilization solution by soaking with 5 mM K 2 PtCl 4 or 5 mM UO 2 (CH 3 COO) 2 for 3–4 h before flash-freezing. Crystallization of PafA Cglu was carried out at a protein concentration of 15–20 mg ml −1 at 4 °C. 2 μl of protein was mixed with 1 μl of reservoir solution (0.1 M CHES-NaOH, pH 9.0, 200 mM Li 2 SO 4 and 22 % (v/v) PEG-4000). Before flash freezing, crystals were stabilized by adding 20% PEG-400. Soaking of PafA crystals with ADP was performed in cryo-stabilization solution with 5 mM ADP for 30 min. Data collection and structure determination The structure of Dop was solved using Pt and uranyl acetate derivatives, whereas PafA was solved via molecular replacement with the Dop structure. Data sets of both Dop Acel and PafA Cglu were collected at beamline X06SA of the Swiss Light Source (Paul Scherrer Institute, Villigen, Switzerland). For data indexing and integration, X-ray detector software (XDS) [25] was used. Scaling and merging of diffraction data as well as calculation of structure factor amplitudes was performed with the CCP4 program SCALA. Locations of Pt and uranyl acetate sites in Dop Acel were determined with programs from the SHELX software package [26] using single- wavelength anomalous dispersion (SAD). Initial phases were obtained using AUTOSOL of the Phenix package [27] , [28] . A preliminary model was generated using BUCCANEER [29] and manually completed and corrected in COOT [30] . Manual rebuilding was alternated with refinement with phenix.refine [28] . To obtain the preliminary model of PafA Cglu , molecular replacement was performed using the program PHASER with Dop Acel as a search model. The 2Fo–Fc maps were of good quality ( Supplementary Fig. S10 ) except for residues 36–80 of Dop and residues 26–31 of PafA; these regions were omitted from the final model. Structures of ATP and ADP ligands for Dop and PafA, respectively, were built into difference Fourier maps obtained by refining the structures of apo enzymes against data obtained from nucleotide-soaked crystals. For PafA, only the ADP-bound structure is presented here because of better diffraction properties. Following refinement of the nucleotides, additional density was interpreted as coordinated Mg 2+ ions. In one of the two copies of PafA in the asymmetric unit of the crystal, the di-phosphate was modelled with two alternative conformations, but only the major one is discussed in the text. Structure determination of enzyme–nucleotide complexes was carried out via COOT and phenix.refine. Molecular graphics representations were created using the software PyMOL ( http://www.pymol.org/ ). Accession codes: Coordinates and structure factors for Dop, Dop ATP and PafA ADP have been deposited in the Protein Data Bank under the accession codes 4B0R , 4B0S and 4B0 T , respectively. How to cite this article: Özcelik, D. et al . Structures of Pup ligase PafA and depupylase Dop from the prokaryotic ubiquitin-like modification pathway. Nat. Commun. 3:1014 doi: 10.1038/ncomms2009 (2012).